Cleavage-based signal amplification of RNA RNA detection has become an integral part of current biomedical research. Up to now, the reverse transcription–PCR has been the most practical method to detect mRNA targets. However, RNA detection by reverse transcription–PCR requires sophisticated equipment and it is highly sensitive to contamination with genomic DNA. Here we report a new isothermal reaction to simultaneously amplify and detect RNA, based on cleavage by DNAzyme and signal amplification. Cleavage-based signal amplification of RNA cannot be contaminated by genomic DNA and is suitable for the detection of both mRNA and microRNA targets, with high specificity and sensitivity. Moreover, the detection results can be reported in a colorimetric or real-time fluorometric way for different detection purposes. RNAs, including messenger RNA and microRNA (miRNA) are very important research targets because of their essential role in living cells. mRNA is a class of RNA molecules encoding the genetic code of DNA, which is eventually translated into protein by ribosome. miRNA is another class of RNA, which is a short ribonucleic acid molecule (18–25 nucleotides), involved in gene silencing. RNA detection has become an important part of current biomedical research, because it is considered a signature for pathogen identification [1] and its expression profile is linked with disease pathogenesis [2] , allowing for biomarker identification [3] . Thus, RNA as a target of interest has attracted a lot of attention from scientific community, because of their great value in medical diagnostics [4] , drug discovery [5] , disease pathophysiology [6] , biochemical pathways [7] and microbial identification [8] . This expansion of interest in studying RNA has generated demand for its accurate and sensitive detection. Several methods for RNA detection have been developed, ranging from simple to complex and multi-step procedures. Among them, reverse transcription–PCR (RT–PCR) [9] is the most sensitive and practical method to detect mRNA targets. However, a main limitation of RT–PCR is its high sensitivity to contamination with genomic DNA. Likewise, miRNA is too short to be amplified by PCR directly, which makes the PCR design very sophisticated [10] , [11] . Thermal cycling of the PCR technique imposes instrumental constraints, limiting the technique to a laboratory setting, and dual-labelled fluorescent probes, such as Taqman probes [12] , are usually needed to determine the specificity of amplification. Therefore, isothermal amplification of RNA, such as nucleic acid sequence-based amplification [13] , [14] , [15] , rolling-cycle amplification [16] , [17] and loop-mediated isothermal amplification [18] , [19] have emerged as alternative amplification techniques. As the above mentioned reactions can be preceded at a constant temperature, there is no need of specialized instruments for RNA detection, and in addition, they have potential for ‘on-site’ testing. However, isothermal amplifications and PCR reactions are usually based on template replication, which increases the risk of cross-contamination and results in false-positive results. Amplification of RNA-induced signals rather than the RNA sequence itself is a better choice to deal with the problem [10] , [20] . A new isothermal reaction to simultaneously amplify and detect RNA based on the cleavage by DNAzyme and signal amplification is reported herein. DNAzymes are catalytic single-stranded DNAs that can be obtained through in-vitro selection [21] , [22] , [23] , [24] , [25] . Two kinds of catalytic DNA sequences, RNA-cleaving DNAzyme (10–23) [26] , [27] and G-quadruplex horseradish peroxidase-mimicking DNAzyme (PW17) [28] , [29] , [30] were applied in our research. The 10–23 RNA-cleaving DNAzyme has been reported to cleave any purine–pyrimidine (RY) junction under simulated physiological conditions [26] ; hence, it was applied in our strategy for the cleaving of target RNA molecule to initiate the following exponential amplification. Furthermore, a special DNAzyme adopting a G-quadruplex structure has been found to exhibit peroxidase-like activity in the presence of hemin; thus, it was also utilized for signal amplification in our method. Recently, this DNAzyme has been explored for the design of various colorimetric or chemiluminescent assays [31] , [32] . The principle of cleavage-based RNA amplification is illustrated in Fig. 1 . The 10–23 DNAzyme, consisting of two binding arms that are complimentary to the target RNA sequence, is used as a probe to bind RNA substrate specifically, where the catalytic core of DNAzyme can cleave the scissile dinucleotide junction. The forward-cleaved RNA fragment, which hybridize with DNAzyme after cleavage, consequently serves as a primer for mesophilic DNA polymerase to replicate the sequence of DNAzyme, and extension of the RNA primer yields double-stranded nucleic acids. A short DNA fragment that contains the recognition site of a nicking endonuclease (purple fragment, Fig. 1 ) is designed at the 5′-end of the 10–23 DNAzyme. Cleavage on double-stranded DNA by nicking enzyme generates a new site for the initiation of extension. A short, single-stranded DNA can be displaced when DNA polymerase carries out the extension. Extension on the template again yields a double-stranded domain that has a recognition site for nicking endonucleases. Hence, extension, cleavage and strand displacement can be repeated continuously in cycles and can release a large amount of short DNA sequences that can trigger the following signal-amplification cascade. 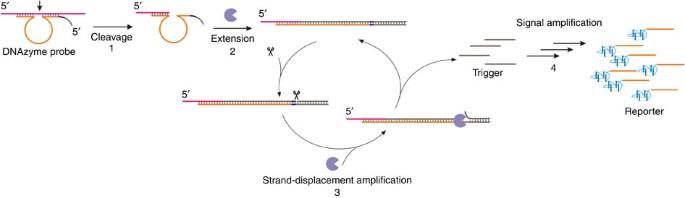Figure 1: Strategy to realize cleavage-based RNA amplification. (1) Site-specific cleavage of target RNA substrate by 10–23 DNAzyme. (2) Extension of cleaved RNA primer to yield double-stranded DNA containing recognition site for nicking enzyme. (3) Strand-displacement amplification releasing single-stranded DNA product that triggers the following signal amplification cascade. (4) Signal amplification creating large amount of G-quadruplex horseradish peroxidase-mimicking DNAzymes, reporting RNA detection. Figure 1: Strategy to realize cleavage-based RNA amplification. (1) Site-specific cleavage of target RNA substrate by 10–23 DNAzyme. (2) Extension of cleaved RNA primer to yield double-stranded DNA containing recognition site for nicking enzyme. (3) Strand-displacement amplification releasing single-stranded DNA product that triggers the following signal amplification cascade. (4) Signal amplification creating large amount of G-quadruplex horseradish peroxidase-mimicking DNAzymes, reporting RNA detection. Full size image Here we show that cleavage-based RNA amplification could only be initiated by the modified 10–23 DNAzyme. Released DNA fragment could then trigger an autonomous signal-amplification cascade; three strand-displacement amplification reactions are linked together to create a large amount of functional G-quadruplexes, which could report the presence of the RNA target through colorimetric reaction or real-time fluorescent tracking. This reaction cannot be contaminated by genomic DNA; hence, it is suitable for the detection of both mRNA and miRNA targets with high specificity and sensitivity. The cleavage and extension of RNA To test the feasibility of cleavage-based RNA amplification, Flag mRNA (57 nt in length) was selected as a target for detection, in which an AU dinucleotide junction was designated as the cleaving site ( Fig. 2a ). According to defined target sequence, the corresponding 10–23 DNAzyme Cat was designed. It contained a catalytic core flanked by two substrate-recognition binding arms (16 nt left and 10 nt right as shown in Fig. 2a ). The left binding arm of Cat was designed to be long enough to retain the cleaved forward RNA fragment on the DNAzyme for the following extension by DNA polymerase. The catalytic ability of DNAzyme Cat was verified by using the 5′-P 32 -labelled Flag mRNA as a substrate in the cleaving reaction, and a clear band of cleavage with predicted length can be seen in polyacrylamide gel (PAGE) analysis (lane 2; Fig. 2b ). However, extension on the forward-cleaved RNA was not detected after the addition of mesophilic DNA polymerase (lane 3; Fig. 2b ). It was speculated that the 10–23 DNAzyme cleaved the RNA phosphodiester bond to yield a forward fragment with the 2′, 3′ cyclic phosphate group, which blocked the extension of RNA primer at the 3′-end by DNA polymerase (I; Fig. 2a ). Therefore, 3′-phosphatase, a T4 polynucleotide kinase (PNK) that is known to add a phosphate group to the 5′-hydroxyl ends of both RNA and DNA, was added to remove the 2′, 3′ cyclic phosphate group [33] (II; Fig. 2a ). As PNK-treated RNA primer still could not be extended by DNA polymerase (lane 4; Fig. 2b ), it was concluded that mismatching at 3′-end of the primer (III; Fig. 2a ) inhibited the replication by DNA polymerase, as with perfect-matched template mCat ( Fig. 2c ), and the same RNA primer was shown to be fully extended (51 nt as expected on lane 6; Fig. 2b ). Therefore, the first nucleotide ‘A’ in the catalytic core of the 10–23 DNAzyme from the 5′-end was replaced by ‘T’ to make the cleavage-based RNA-amplification strategy feasible. Nevertheless, modification in the catalytic core sequence of the 10–23 DNAzyme usually results in loss of RNA-cleaving catalytic ability [34] , [35] , [36] . 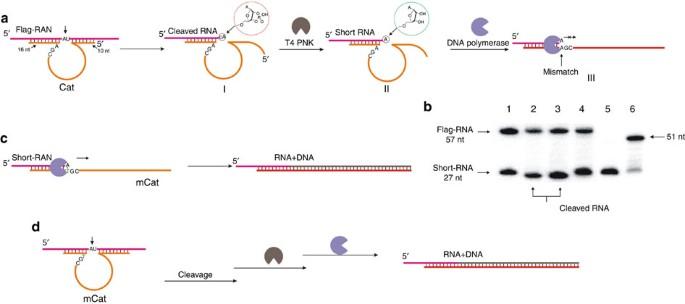Figure 2: Cleavage of DNAzyme on RNA substrate and extension of RNA primer by DNA olymearase. (a) Flag-RNA (5′-GGAGGACGAAAUGGACUACAAGGACGAUGACGAUAAGCAGCUGCGUAACUCUAAAAA-3′; italic: cleaving site; underscore: binding domain) was cleaved by 10–23 DNAzymeCat(5′-CTTATCGTCAGGCTAGCTACAACGACGTCCTTGTAGTCCAT-3′, boldface: catalytic core; underscore: binding arms) to yield a forward RNA fragment with 2′, 3′ cyclic phosphate group on 3′-end (I); PNK treatment removed the cyclic phosphate group (II); DNA polymerase cannot replicate the RNA primer with a mismatch at 3′-end (III). (b) PAGE analysis of cleaving and extension reactions. Lane 1: two markers, 5′-32P-labelled Flag-RNA (57 nt) andin-vitrotranscribed forward RNA fragment short-RNA (27 nt); lane 2: cleavage of32P-labelled Flag-RNA by DNAzymeCat. Cleaved product has slightly faster mobility because of the presence of 2′, 3′ cyclic phosphate group at the 3′-end; lane 3: extension catalysed by Bsm DNA polymerase (Fermentas) after cleavage; lane 4: extension by DNA polymerase after cleavage and PNK treatment; lane 5: marker, 5′-labelled short-RNA (27 nt); lane 6: extension of 5′-P32-labelled short-RNA primer on modified templatemCatby DNA polymerase (as shown inc). (c) Short-RNA extended by DNA polymerase on a modified templatemCat, which has only one mutation (green colour) in comparison with the sequence ofCat. (d) Experiment to evaluate the modified DNAzymemCat(5′-CTTATCGTCAGGCTAGCTACAACGTCGTCCTTGTAGTCCAT-3′, boldface: catalytic core; underscore: binding arms; italic: A to T substitution). Figure 2: Cleavage of DNAzyme on RNA substrate and extension of RNA primer by DNA olymearase. ( a ) Flag-RNA (5′-GGAGGACGAA AUGGACUACAAGGACG A U GACGAUAAG CAGCUGCGUAACUCUAAAAA-3′; italic: cleaving site; underscore: binding domain) was cleaved by 10–23 DNAzyme Cat (5′- CTTATCGTCA GGCTAGCTACAACGA CGTCCTTGTAGTCCAT -3′ , boldface: catalytic core; underscore: binding arms) to yield a forward RNA fragment with 2′, 3′ cyclic phosphate group on 3′-end ( I ); PNK treatment removed the cyclic phosphate group ( II ); DNA polymerase cannot replicate the RNA primer with a mismatch at 3′-end ( III ). ( b ) PAGE analysis of cleaving and extension reactions. Lane 1: two markers, 5′- 32 P-labelled Flag-RNA (57 nt) and in-vitro transcribed forward RNA fragment short-RNA (27 nt); lane 2: cleavage of 32 P-labelled Flag-RNA by DNAzyme Cat . Cleaved product has slightly faster mobility because of the presence of 2′, 3′ cyclic phosphate group at the 3′-end; lane 3: extension catalysed by Bsm DNA polymerase (Fermentas) after cleavage; lane 4: extension by DNA polymerase after cleavage and PNK treatment; lane 5: marker, 5′-labelled short-RNA (27 nt); lane 6: extension of 5′-P 32 -labelled short-RNA primer on modified template mCat by DNA polymerase (as shown in c ). ( c ) Short-RNA extended by DNA polymerase on a modified template mCat , which has only one mutation (green colour) in comparison with the sequence of Cat . ( d ) Experiment to evaluate the modified DNAzyme mCat (5′- CTTATCGTCA GGCTAGCTACAACG T CGTCCTTGTAGTCCAT -3 ′, boldface: catalytic core; underscore: binding arms; italic: A to T substitution). Full size image Fortunately, the modified 10–23 DNAzyme mCat still keep the cleaving ability, even though the mutant site was located in the highly conserved position for the 10–23 catalytic activity [34] ( Fig. 2d ). Modified 10–23 DNAzyme was found to be quite an efficient RNA-cleaving DNAzyme, with a k obs of 0.018 min −1 ( Supplementary Fig. S1 ), which was relatively lower than that of the unmodified DNAzyme Cat ( k obs of 0.198 min −1 ; Supplementary Fig. S1 ). In 1 h, more than half of the RNA substrates were cleaved (lane 2; Supplementary Fig. S2 ) and forward-cleaved fragments were successfully extended by DNA polymerase (lane 4; Supplementary Fig. S2 ). However, treatment with PNK that removes the 2′, 3′ cyclic phosphate group on the RNA primer was indispensable for extension on cleaved RNA by DNA polymerase (lane 3; Supplementary Fig. S2 ). Signal amplification To induce signal amplification after cleavage of RNA target, extra sequence that contains both recognition site of nicking endonuclease and a specific antisense sequence, namely Ts , was added to the 5′-end of mCat to construct an fCat probe ( Fig. 3a ), to serve as the initiator of signal amplification. Catalytic ability of fCat was similar to mCat , and the cleaved RNA fragment was extended by DNA polymerase to yield a double-stranded product (step 2; Fig. 3a ) after the 2′, 3′ cyclic phosphate group has been removed by PNK (lane 2–4, Supplementary Fig. S3 ). 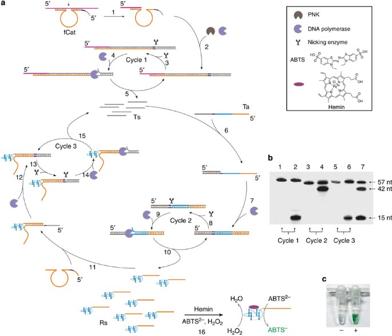Figure 3: The principle of cleavage-based RNA amplification and verification experiments. (a) Scheme of cleavage-based RNA amplification. Step 1: cleavage of RNA substrates by DNAzymefCat, which contains sequence ofmCat(orange), recognition site of nicking enzyme (purple) and antisense sequence ofTs(grey). Step 2: treatment with PNK removes the cyclic phosphate group of RNA primer. The resulting RNA primer is then extended by DNA polymerase. Step 3–5 (cycle 1): first strand-displacement amplification yields Trigger sequencesTs. Step 6: hybridization betweenTsand probeTa, which consists of four parts: the antisense sequence ofTs(grey), recognition site of nicking endonuclease (purple), antisense sequence of DNAzyme (blue) and partial sequence offCatcatalytic core (red) from 3′- to 5′-end. Step 7–10 (cycle 2): second strand-displacement amplification yields single-stranded DNA product (Rs), which contains two parts: peroxidase-mimicking DNAzyme sequence (blue) and antisense sequence of partialfCatcatalytic core (red). Step 11: hybridization betweenRsandfCat. Step 12–15 (cycle 3): third strand-displacement amplification yieldsTssequences. Step 16: colorimetric reaction after amplification by adding hemin, ABTS and H2O2. (b) PAGE analysis of strand-displacement amplification of cycle 1–3. Lane 1: PAGE analysis of step 2 by adding [α-32P]dCTP into the reaction mixture; lane 2: PAGE analysis of step 2–5; lane 3: PAGE analysis of step 6–7 by using [α-32P]dCTP; lane 4: PAGE analysis of step 6–10; lane 5: PAGE analysis of step 11–12; lane 6: PAGE analysis of step 11–15; lane 7: three markers, 5′-32P-labelled Flag-RNA (57 nt),Rs(42 nt),Ts(15 nt). (c) The photograph of colorimetric result; ‘+’ including 10−8mol RNA target; ‘−’ negative control (a sample of H2O). Figure 3: The principle of cleavage-based RNA amplification and verification experiments. ( a ) Scheme of cleavage-based RNA amplification. Step 1: cleavage of RNA substrates by DNAzyme fCat , which contains sequence of mCat (orange), recognition site of nicking enzyme (purple) and antisense sequence of Ts (grey). Step 2: treatment with PNK removes the cyclic phosphate group of RNA primer. The resulting RNA primer is then extended by DNA polymerase. Step 3–5 (cycle 1): first strand-displacement amplification yields Trigger sequences Ts . Step 6: hybridization between Ts and probe Ta , which consists of four parts: the antisense sequence of Ts (grey), recognition site of nicking endonuclease (purple), antisense sequence of DNAzyme (blue) and partial sequence of fCat catalytic core (red) from 3′- to 5′-end. Step 7–10 (cycle 2): second strand-displacement amplification yields single-stranded DNA product ( Rs ), which contains two parts: peroxidase-mimicking DNAzyme sequence (blue) and antisense sequence of partial fCat catalytic core (red). Step 11: hybridization between Rs and fCat . Step 12–15 (cycle 3): third strand-displacement amplification yields Ts sequences. Step 16: colorimetric reaction after amplification by adding hemin, ABTS and H 2 O 2 . ( b ) PAGE analysis of strand-displacement amplification of cycle 1–3. Lane 1: PAGE analysis of step 2 by adding [α- 32 P]dCTP into the reaction mixture; lane 2: PAGE analysis of step 2–5; lane 3: PAGE analysis of step 6–7 by using [α- 32 P]dCTP; lane 4: PAGE analysis of step 6–10; lane 5: PAGE analysis of step 11–12; lane 6: PAGE analysis of step 11–15; lane 7: three markers, 5′- 32 P-labelled Flag-RNA (57 nt), Rs (42 nt), Ts (15 nt). ( c ) The photograph of colorimetric result; ‘+’ including 10 −8 mol RNA target; ‘−’ negative control (a sample of H 2 O). Full size image Furthermore, a nicking endonuclease, which could recognize specific nucleotide sequences in double-stranded DNA and cleave only one strand, was added into the reaction to obtain nicked DNA (step 3, Fig. 3a ). Subsequently, the forward-cleaved DNA strand was extended by using DNA polymerase (step 4, Fig. 3a ), and the short DNA sequence Ts behind the nicking site was released, owing to the strand-displacement property of DNA polymerase (step 5, Fig. 3a ), which triggered the downstream signal amplification. To validate strand-displacement amplification (cycle 1; Fig. 3a ) after cleavage, isotope-labelled [α- 32 P]dCTP was added in two parallel replication reactions, except nicking endonuclease in one of them. A band that corresponds in size to the cleaved fragment Ts appeared on denaturing PAGE gel when nicking enzyme was added into the reaction (lane 1–2; Fig. 3b ). In our strategy of signal amplification, released DNA strand Ts was hybridized to a single-stranded DNA probe Ta , which had been already added into the reaction mixture. Ta consisted of four parts from the 3′- to 5′-end: (1) the antisense sequence of the trigger Ts (grey); (2) the recognition site for nicking endonuclease (purple); (3) the antisense sequence of PW17 horseradish peroxidase-mimicking DNAzyme (blue); and (4) the partial sequence of fCat catalytic core (red). Once the trigger sequence Ts was captured by the probe Ta , DNA polymerase and nicking endonuclease in the reaction would process on the Ts – Ta duplex hybrid alternatively, to yield a large amount of single-stranded DNA product Rs (cycle 2; Fig. 3a ), which could fold into a G-quadruplex structure with a tail on the 3′-end. G-quadruplex can bind hemin to exhibit peroxidase-like activity and act as a reporter of RNA amplification. The signal amplification could not be stopped at this step, because the tail of Rs hybridized with an unreacted fCat to initiate a new strand-displacement amplification (cycle 3; Fig. 3a ). Upon hybridization with DNAzyme, the tail of Rs was extended by using DNA polymerase to yield a duplex product containing a nicking-enzyme recognition site. Repeated cleavage, extension and displacement resulted in linear amplification of a short sequence Ts , which was fed into cycle 2 again and resulted in exponential amplification. The final result of signal amplification was the accumulation of the G-quadruplex product Rs . Hemin was added into the reaction mixture after amplification, and DNAzyme oxidized the colourless ABTS (2,2′-azino-bis(3-ethylbenzthiazoline-6-sulphonic acid)) into a green-coloured product in the presence of H 2 O 2 . Thus, detection result could be read through direct observation of colour change in the reaction mixture. Each strand-displacement amplification reaction (cycle 1–3) in the whole signal-amplification process was visualized using gel electrophoresis, which revealed the presence of both extension and cleavage bands ( Fig. 3c ). Endpoint colorimetric detection of target mRNA was realized by adding hemin, ABTS and H 2 O 2 in the tube of amplification reaction, as illustrated in Fig. 3c . The qualitative result could be read directly by the naked eyes. Colorimetric detection The optimum concentrations of DNA polymerase, PNK, nicking enzyme and probes for RNA amplification were found to be 0.125, 0.25 and 0.125 U μl −1 , and 0.25 μM, respectively, in a reaction volume of 20 μl. The best temperature for amplification was 37 o C. Under optimal conditions, Flag mRNA target could be detected colorimetrically in the range of 1 fmol–100 pmol by visual appreciation of reaction tubes after adding hemin, ABTS and H 2 O 2 ( Fig. 4a ). To check the potential influence of genetic DNA on RNA detection, same amount of single-stranded and double-stranded DNA, encoding identical sequence with Flag-RNA, were analysed (tube c and d; Fig. 4b ). Colorimetric results have indicated that the genetic DNA could not induce amplification. To evaluate specificity of the proposed RNA assay, 0.3 ng of total RNA from HepG2 cells was added into the sample, which imitates a real-life RNA assay. Colorimetric result of the sample that contained both target RNA and RNA of the HepG2 cell was distinctively different from the negative control reaction, in which RNA of the HepG2 cells was added (tube e and f; Fig. 4b and Supplementary Fig. S4 ). High specificity of cleavage-based RNA detection is attributed to the DNAzyme probe that can only cleave at the right dinucleotide junction of RNA substrates based on the strict Watson–Crick base-pairing rule. 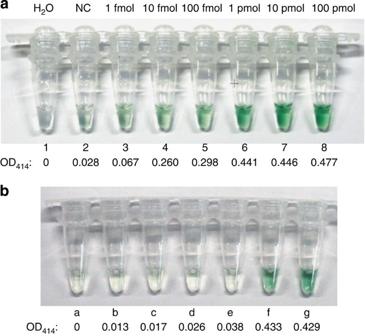Figure 4: Sensitivity and specificity of colorimetric RNA detection. (a) Colorimetric detection of flag-RNA with different concentrations of RNA targets. NC (negative control): detection reaction without RNA target; (b) specificity of cleavage-based RNA assay based on colorimetric reaction. Tube a: H2O; tube b: NC (negative control) detection reaction without RNA target; tube c: 200 fmol of single-stranded DNA, which encodes the same genetic information as Flag-RNA; tube d: 200 fmol of double-stranded DNA which encodes the genetic information of Flag-RNA; tube e: 0.3 ng of total RNA extracted from HepG2 cell; tube f: 200 fmol of target RNA and 3 ng of total RNA extracted from HepG2 cell; tube g: PC (positive control) reaction with 200 fmol target RNA. OD414: optical density at 414 nm. Figure 4: Sensitivity and specificity of colorimetric RNA detection. ( a ) Colorimetric detection of flag-RNA with different concentrations of RNA targets. NC (negative control): detection reaction without RNA target; ( b ) specificity of cleavage-based RNA assay based on colorimetric reaction. Tube a: H 2 O; tube b: NC (negative control) detection reaction without RNA target; tube c: 200 fmol of single-stranded DNA, which encodes the same genetic information as Flag-RNA; tube d: 200 fmol of double-stranded DNA which encodes the genetic information of Flag-RNA; tube e: 0.3 ng of total RNA extracted from HepG2 cell; tube f: 200 fmol of target RNA and 3 ng of total RNA extracted from HepG2 cell; tube g: PC (positive control) reaction with 200 fmol target RNA. OD 414 : optical density at 414 nm. Full size image Real-time fluorescence assay Colorimetric detection is a very convenient way to realize on-site test for RNA target for qualitative result as well as quantitative analysis of target RNA, which is possible by measuring ultraviolet absorption intensities of the colorimetric reaction. However, to achieve more accurate quantitative detection of RNA targets, it is better to monitor the progress of amplification reaction on real-time basis. Therefore, probe Ta in our previous signal-amplification strategy was substituted by probe Tb ( Fig. 5a ), which encode the antisense sequence for another G-quadruplex ‘Hum21’, which is a mimic of human telomeric sequence. Triphenylmethane dyes, such as malachite green and crystal violet, can bind to part of Hum21 G-quadruplex, which results in greatly enhanced fluorescence intensities [37] . Under optimal reaction conditions, malachite green was found to be a much better dye than crystal violet for Hum21 G-quadruplex in terms of the fluorescence enhancement, and no effect on signal-amplification reaction was noticed after the addition of malachite green. When a new probe Tb was applied in the detection strategy, Hum21 G-quadruplex was amplified, and after binding with malachite green an increase of fluorescence was detected with the progress of reaction. Unlike Taqman probe, which is a fluorophore-modified oligonucleotide, relatively low-cost malachite green dye can decrease the cost of real-time RNA detection considerably. Real-time isothermal cleavage-based RNA detection is very easy to realize either on a fluorescence microplate reader or a real-time PCR machine. The fluorescence curves of the reaction revealed that amplification proceeded in exponential fashion ( Fig. 5b ). Threshold time T T is defined as the time when fluorescent intensity exceeds an arbitrary threshold, which is an analogy to the threshold cycle ( C T ) in real-time PCR analysis. The T T values are linearly dependent on the logarithm of the amount of target mRNA in a range of 1 nM to 10 fM ( Fig. 5b ). The correlation equation is T T =−3.528 lg(C RNA )+32.087 ( R 2 =0.969), and the detection limitation is 69.2 aM ( Fig. 5c ). Moreover, the whole detection process was conducted in a one-step manner without opening the tube during the whole process, which is common in a two-step RT–PCR reaction. This would decrease the possibility of cross-contamination in the operation and make cleavage-based RNA amplification feasible in a high-throughput set up. 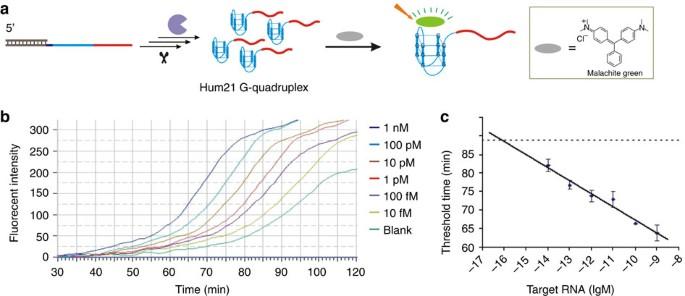Figure 5: Real-time fluorometric detection of cleavage-based RNA amplification. (a) Scheme of the strategy to realize real-time fluorescent detection of RNA target based on fluorescence signal. ProbeTbis the same as probeTa, except the blue part, which was changed into the antisense sequence of Hum21 G-quadruplex. (b) Real-time fluorescence curve of RNA detection. Blank: detection reaction without any RNA target. (c) Threshold timeTTwas plotted against the concentration of target RNA (CRNA). The solid line indicates linear least squares fitting between 1 nM and 10 fM of RNA target, and their formulation isTT=−3.528 lg(CRNA)+32.087 (R2=0.969). Error bar represents the variation between duplicate experiments. The perforated line indicates averageTTvalue of negative controls (blank inc). Detection limit was 69.2 aM of RNA targets by calculation from the intersection of both lines. Figure 5: Real-time fluorometric detection of cleavage-based RNA amplification. ( a ) Scheme of the strategy to realize real-time fluorescent detection of RNA target based on fluorescence signal. Probe Tb is the same as probe Ta , except the blue part, which was changed into the antisense sequence of Hum21 G-quadruplex. ( b ) Real-time fluorescence curve of RNA detection. Blank: detection reaction without any RNA target. ( c ) Threshold time T T was plotted against the concentration of target RNA (C RNA ). The solid line indicates linear least squares fitting between 1 nM and 10 fM of RNA target, and their formulation is T T =−3.528 lg(C RNA )+32.087 ( R 2 =0.969). Error bar represents the variation between duplicate experiments. The perforated line indicates average T T value of negative controls (blank in c ). Detection limit was 69.2 aM of RNA targets by calculation from the intersection of both lines. Full size image Enhanced green fluorescent protein (eGFP) mRNA extracted from cancer cells was selected as the target to verify our method in a real-world application, because mRNA in cancer cells could easily be verified by expression of relative protein, and total RNA extracted from untransfected cells were used as negative control to investigate the specificity of our method. On the basis of our previous results of cleaving eGFP mRNA by using 10–23 DNAzyme [38] , we have selected the AU dinucleotide junction at 527–528 nt of eGFP mRNA as the cleaving site. And cleavage of eGFP RNA fragment (79 nt) by DNAzyme was verified by PAGE analysis ( Supplementary Fig. S5 ). The eGFP-expressing Hela cells were examined under a fluorescence microscope ( Supplementary Fig. S6 ). Different concentration of total RNA extracted from the eGFP-expressing Hela cells were detected by our cleavage-based signal-amplification system ( Supplementary Fig. S7 ) and RT–PCR assay ( Supplementary Fig. S8 ), whereas total RNA extracted from untransfected Hela cells was used as negative control. We got similar real-time fluorescence curve as illustrated in Fig. 5c , and eGFP mRNA obtained from 3,000 transfected Hela cells could be detected. Sensitivity of cleavage-based signal amplification was at least one order of magnitude lower than that of the RT–PCR reaction and specificity was not comparable to that of the RT–PCR, but this method is still promising enough for real-world detection in respect of easy operation, no genomic DNA contamination and isothermal amplification. Substrate-scope investigation In theory, cleavage-based amplification could be applied in detection of any RNA target if it was cleaved by the DNAzyme probe. The original 10–23 DNAzyme can cleave almost any target RNA that contains a purine–pyrimidine junction (R ↓ Y, R=A or G; Y=U or C). However, the RNA substrate with AU junction has only been successfully cleaved by modified 10–23 DNAzyme probe, in which the first nucleotide A in the catalytic core was modified with T to make the cleaved RNA fragment complementary with the DNAzyme sequence at 3′-end. To explore the scope of this strategy to RNA with other purine–pyrimidine junctions, cleavage reactions of four possible substrates with different RY junctions were examined using the corresponding modified 10–23 DNAzymes ( Fig. 6a ). The electrophoresis results of cleavage reaction are illustrated in Fig. 6b . Only two types of the purine–pyrimidine junction, AU and GU, could be cleaved by the corresponding modified DNAzymes. This indicated that the cleavage-based RNA detection method could be applied to RNA sequences with RU (R=A or G) junction, which occurs with high frequency as one repeat in every 8 bp. More importantly, threshold requirement of cleavage-based signal amplification of RNA could be satisfied very easily, and length of RNA was not found to be a limiting factor for application scope of this method if the RNA target was long enough to be cleaved by DNAzyme at the right position. 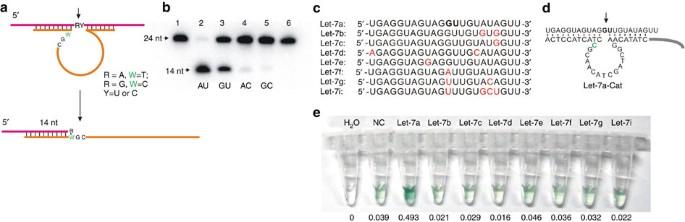Figure 6: Substrate-scope investigation. (a) Cleavage of four possible purine–pyrimidine junctions by modified 10–23 DNAzyme. (b) Cleavage of different RNA substrates with corresponding DNAzymes. Lanes 1 and 6: marker of flag-RNA (24 nt) and cleaved fragment (14 nt); lane 2–5: cleaving reactions of RNA substrate with AU, GU, AC, GC dinucleotide junctions by corresponding modified DNAzymes. (c) Sequence information of miRNA Let-7a–g and Let-7i. Nucleobases of other family members, which differ from Let-7a are marked in red. (d) DNAzyme probeLet-7a-Catwas designed to initiate the cleavage-based assay of miRNAlet-7aspecifically. Arrow points the cleaving site of Let-7a by DNAzyme. (e) Colorimetric detection of 200 fmol of miRNALet-7a-gandLet-7iwith DNAzyme probeLet-7a-Cat. NC (negative control): detection reaction without any RNA target. OD414: optical density at 414 nm. Figure 6: Substrate-scope investigation. ( a ) Cleavage of four possible purine–pyrimidine junctions by modified 10–23 DNAzyme. ( b ) Cleavage of different RNA substrates with corresponding DNAzymes. Lanes 1 and 6: marker of flag-RNA (24 nt) and cleaved fragment (14 nt); lane 2–5: cleaving reactions of RNA substrate with AU, GU, AC, GC dinucleotide junctions by corresponding modified DNAzymes. ( c ) Sequence information of miRNA Let-7a–g and Let-7i. Nucleobases of other family members, which differ from Let-7a are marked in red. ( d ) DNAzyme probe Let-7a-Cat was designed to initiate the cleavage-based assay of miRNA let-7a specifically. Arrow points the cleaving site of Let-7a by DNAzyme. ( e ) Colorimetric detection of 200 fmol of miRNA Let-7a-g and Let-7i with DNAzyme probe Let-7a-Cat . NC (negative control): detection reaction without any RNA target. OD 414 : optical density at 414 nm. Full size image To validate the application of detection system for short-RNA target, miRNA Let-7a ( Fig. 6c ) was selected as the target [39] , which is only 22 nt long and contained a GU dinucleotide junction in the middle. The Let - 7a - Cat probe was designed to cleave Let-7a, specifically at the GU junction ( Fig. 6d ). Colorimetric assay of miRNA Let-7a was almost the same as for mRNA, except the design of the DNAzyme probe sequence. Member of the Let-7 miRNA family (Let-7a–g and i) was selected as the model system to evaluate the specificity of our cleavage-based RNA assay because of their high sequence homology ( Fig. 6c ). Colour signal produced by Let-7a could easily be distinguished from other Let-7 families ( Fig. 6e ), in which some members have only one base difference from Let-7a, such as Let-7e and Let-7f ( Fig. 6c ). Real-time fluorescence assay of the Let-7a miRNA family with Let - 7a - Cat and Tb probes was consistent with the colorimetric result, which verified the high specificity of our cleavage-based detection method ( Supplementary Fig. S9 ). Difference of threshold time Δ T T between Let-7a and the closest one of Let-7 family members was more than 10 min on real-time fluorescence curves ( Supplementary Fig. S9 ). The cleavage-based amplification scheme described here appears to have several promising features for research and diagnostic applications as follows: (1) isothermal nature of this method makes it more applicable than RT–PCR, because neither thermally stable enzyme nor sophisticated instrumentation is required to conduct this assay. (2) Here the amplification is based on cleavage of the target RNA rather than template replication; thus, RNA target or its encoded genetic information is not propagated but decayed after the process of amplification, lowering the risk of cross-contamination from amplicons. (3) Established assay offers high specificity and high sensitivity, as the recognition of RNA substrate by the binding arms (>20 nt) of DNAzyme according to Watson–Crick base pair is the first safeguard to specificity. Cleavage of the RNA target at the right dinucleotide junction to initiate amplification is the second warrant of high specificity. Moreover, DNA sequence encoding the same genetic information as the RNA target is not able to initiate amplification, because 10–23 DNAzyme cannot cleave the DNA substrates. Therefore, contamination with genomic DNA is not a problem of the cleavage-based RNA detection method. Here we have combined three strand-displacement amplifications together as a chain of reactions, which provides more than 10 6 -fold amplifications within 2 h. 4) Flexibility of reaction with which the signal amplification can be triggered and elaborated into multiple reactions to obtain either colorimetric or fluorescent results for different detection purposes. The cleavage-based RNA detection presented here is suitable for use with diverse mRNA and miRNA targets, because the modified 10–23 DNAzyme probes has inherently broad substrate tolerance and high specificity to target RNA. Three strand-displacement amplification reactions linked together in our strategy and achieved highly efficient signal amplification. Introduction of functional G-quadruplex into the amplification strategy as a reporter makes RNA assay a versatile method, which can be realized as ‘on-site’ detection by colorimetric way, or in highly sensitive real-time manner to obtain accurate quantitation based on fluorescence assay. General information T7 RNA polymerase, FastAP Thermosensitive Alkaline Phosphatase (FastAP), T4 PNK), Bsm DNA polymerase, Klenow fragment exo-polymerase and Nb.Bpu10I nicking endonuclease were purchased from MBI Fermentas. NTP and dNTP were purchased from TransGen Biotech (Beijing, China). [γ-32P]ATP, [α-32P]dATP and [α-32P]dCTP were purchased from Furui Biological Engineering (Beijing, China). Hemin was purchased from Alfa Aesar, whereas stock solution was prepared in dimethyl sulphoxide and stored in the dark at −20 °C. ABTS was purchased from Wolsen (Xi an, China); H 2 O 2 was purchased from Bodi Chemical Holding Co., Ltd (Tianjin, China); and all oligonucleotides were purchased from Sangon Biotech (Shanghai, China) and purified by HPLC. RNA transcription RNA substrates were synthesized by RNA transcription using T7 RNA polymerase and a double-stranded DNA template having the following sense sequence 5′-GAATT C TAATACGACTCACTATA- RNA-3′ (italicized letters indicates the promoter sequence for T7 RNA polymerase). A transcription reaction containing 0.5 μM of DNA template, 10 mM of NTP, 1 × T7 RNA polymerase buffer (40 mM Tris–HCl (pH 7.9), 10 mM NaCl, 10 mM dithiothreitol, 6 mM MgCl 2 , 2 mM spermidine) and 1.25 unit per μl RNA polymerase were incubated at 37 °C for 4 h, followed by ethanol precipitation and purification by PAGE. Labelling reaction A reaction mixture containing oligonucleotides with 50 mM Tris–HCl (pH 7.8), 40 mM NaCl, 10 mM MgCl 2 , 1 mg ml −1 BSA, 10 μCi [γ- 32 P]ATP and 10 units of PNK was incubated for 1 h at 37 °C for DNA phosphorylation. The labelled product was purified by 10% denaturing PAGE. Single-stranded DNA could be labelled directly, but RNA substrates obtained by in-vitro transcription must be treated with alkaline phosphatase as follows: RNA was incubated with 0.05 unit per μl FastAP in 10 mM Tris–HCl (pH 8.0), 5 mM MgCl 2 , 100 mM KCl, 0.02% Triton X-100 and 0.1 mg ml −1 BSA at 37 °C for 10 min, and then extracted with phenol–chloroform and recovered by ethanol precipitation. Kinetic analysis of DNAzymes Cleavage reaction containing 20 μM DNAzymes, 100 nM 32 P-labelled Flag-RNA, 10 mM Tris–HCl (pH 8.5), 100 mM KCl, 10 mM MgCl 2 and 0.01 mg ml −1 BSA was incubated at 37 °C. The reaction was stopped after a designated period of time, by adding EDTA (pH 8.0) to a final concentration of 30 mM. Cleavage products were separated by 10% denaturing PAGE and quantified by phosphorimager (PerkinElmer Cyclone Plus Storage Phosphor System). Time courses for each deoxyribozyme were conducted at least twice, using over eight time points for each. The experimental data was fit to the Y=Y max (1-e (− k obst) ) exponential equation using non-linear regression analysis in GraphPad Prism 4, from which the observed rate constant ( k obs ) and maximum cleavage yield ( Y max ) were determined. Cleavage and extension of RNA A cleavage reaction mixture containing 6 μM DNAzymes, 150 nM 5′- 32 P-labelled Flag-RNA, 10 mM Tris–HCl (pH 8.5), 100 mM KCl, 10 mM MgCl 2 and 0.01 mg ml −1 BSA was incubated at 37 °C for 1 h. Afterwards, PNK (0.5 unit per μl) and Bsm polymerase (0.4 unit per μl) were added into the reaction mixture for 30 min. All reactions were analysed by running in a 10% denaturing PAGE. Colorimetric detection Flag-RNA targets were first added into a detection solution to a final volume of 10 μl, containing specified concentrations of targets, 0.25 μM fCat , 0.25 unit per μl PNK, 10 mM Tris–HCl (pH 8.5), 100 mM KCl, 10 mM MgCl 2 and 0.1 mg ml −1 BSA, and incubated at 37 °C for 150 min. Then, 0.25 μM Ta , dNTPs (250 μM), Nb.Bpu10I (0.125 unit per μl) and Klenow exo-polymerase (0.125 unit per μ1) were added to a final volume of 20 μl and incubated for 60 min at 37 °C. Finally, 1.7 μl Tris–HCl (pH 7.3), hemin (1.8 μM), H 2 O 2 (2.1 mM) and ABTS (2.1 mM) were added at 25 °C to the reaction mixture, and colorimetric result was recorded immediately by a digital camera. Real-time fluorescence assay Real-time fluorescence assay was carried out in a 20-μl reaction mixture containing 10 mM Tris–HCl (pH 7.0), 100 mM KCl, 10 mM MgCl 2 , 0.1 mg ml −1 BSA, dNTPs (250 μM), 0.17 unit per μl Nb.Bpu10I, 0.17 unit per μl Bsm DNA polymerase, 0.08 unit per μl PNK, malachite green (15 μmol), 0.25 μM fCat , 0.25 μM Tb and specified concentrations of Flag-RNA targets. The reaction was performed in a real-time PCR system (chanel 4, excitation 600–640 nm, emission 666–740 nm; PikoREAL, Thermo, USA) at 39 °C. Real-time fluorescence intensity was monitored at intervals of 1 min. How to cite this article: Zhao, Y. et al. Cleavage-based signal amplification of RNA. Nat. Commun. 4:1493 doi: 10.1038/ncomms2492 (2013).